Water-induced correlation between single ions imaged at the solid–liquid interface When immersed into water, most solids develop a surface charge, which is neutralized by an accumulation of dissolved counterions at the interface. Although the density distribution of counterions perpendicular to the interface obeys well-established theories, little is known about counterions’ lateral organization at the surface of the solid. Here we show, by using atomic force microscopy and computer simulations, that single hydrated metal ions can spontaneously form ordered structures at the surface of homogeneous solids in aqueous solutions. The structures are laterally stabilized only by water molecules with no need for specific interactions between the surface and the ions. The mechanism, studied here for several systems, is controlled by the hydration landscape of both the surface and the adsorbed ions. The existence of discrete ion domains could play an important role in interfacial phenomena such as charge transfer, crystal growth, nanoscale self-assembly and colloidal stability. The spatial arrangement of ions at solid–liquid interfaces is a problem central to many fields, ranging from electrochemistry [1] to colloidal science [2] , heterogeneous catalysis [3] , surface science [4] or biology [5] . When immersed into a liquid, most solids develop charges at their surface. To maintain electric neutrality, the counterions dissolved in the liquid tend to accumulate close to the solid’s surface, forming an electrostatic double layer (EDL) that counterbalances the solid’s surface charge. The precise structure and spatial distribution of ions in the EDL has been the subject of intense experimental and theoretical research over the last century. At the present time, the most widely used EDL model, the Gouy–Chapman–Stern model (see, for example, Bard and Faulkner [6] ) assumes a dense monolayer of counterions, the Stern or Helmholtz layer (hereafter called Stern layer) adsorbed onto the surface of the solid, followed by a diffuse layer of counterions whose density decays exponentially when moving away from the solid. Most EDL models, including Gouy–Chapman–Stern model, rely on the so-called continuum assumption: ions are modelled as point charges in a continuous dielectric environment. Although routinely verified in the diffuse layer region, these models tend to fall short in the Stern layer region [7] , where the discrete size of ions can no longer be ignored. These difficulties are particularly obvious in highly charged systems [8] , [9] and corrections have been proposed to better account for the complex interactions linking ions, liquid molecules and the surface structure of the solid [10] . Continuum models usually make the implicit assumption that the Stern layer is homogenous, with a uniform ion distribution. This assumption becomes problematic at the nanoscale where most solids exhibit some structure with localized charges and a well-defined hydration landscape that can determine the position and organization of single ions at the interface. Such a complexity is key to many processes such as the folding and function of biomolecules [11] , the accumulation and transfer of charges at the surface of extremophiles [12] , [13] or at the electrodes of solar cells [14] , electro-friction [15] , the nucleation of nanoparticles on surfaces [16] , or the preferential adsorption of a particular type of ion onto minerals [17] . Even at the macroscopic level, intense research is currently dedicated to the synthesis of colloid particles exhibiting non-homogeneous charge distributions at their surface for better controlling the stability or ordering of colloidal solutions [18] . Part of the difficulty in developing suitable models comes from the lack of experimental results. Probing the lateral organization of ions within Stern layers is a challenging task and most results available to date stem either from computer simulations [15] or theoretical developments [19] , [20] . When available, experimental results are typically obtained indirectly [10] or through techniques that require averaging over a large area of the interface [21] , hence implicitly relying on the assumption of a homogeneous Stern layer to provide a precise picture of the position of the ions and the liquid molecules. These difficulties can in principle be overcome by local probe techniques such as atomic force microscopy (AFM). When operated in liquid, AFM is able to investigate solid–liquid interfaces locally, often with atomic- or molecular-level resolution [22] , [23] , [24] , [25] , [26] , [27] , [28] , [29] , [30] , [31] and in the presence of ions [32] , [33] , [34] , [35] , [36] . Studies allowing a clear and unequivocal identification of single ions within a Stern layer are however still sparse, with little information about the formation, stability and dynamics of adsorbed ions at the nanoscale. Here we use AFM to image different hydrated monovalent metal ions adsorbed at the surface of mica in water. We show, with single ion resolution, that the metal ions do not adsorb randomly but form preferentially ordered structures such as rows or geometrical domains due to ion–ion attractive interactions controlled by the water at the interface. The results, confirmed by molecular dynamics (MD) simulations, show that water alone can provide a sufficient driving force to induce order within Stern layers, at least for chaotropic monovalent ions [37] (throughout the paper, we consistently use the concepts of ‘chaotropic’ and ‘kosmotropic’ as defined in ref. 37 ). The key element is the interplay between the local solvation landscape of the solid at the interface and the hydration structure of the ion. Electrostatic interactions induce the adsorption of ions at the Stern layer but do not play any significant role in regulating interactions between monovalent ions within this region. This work presents, to the best of our knowledge, the first direct observation of this correlation mechanism. Significantly, the fact that it occurs between monovalent metal ions at interfaces suggests a common occurrence in natural and synthetic systems. Our findings are confirmed with different types of monovalent ions and also demonstrated on a polar self-assembled monolayer (SAM). The latter is chemically different than mica and, although only weakly charged, provides an appropriate hydration landscape that allows for the formation of ionic structures stable enough to be observed by AFM. The generality of the effect suggests that it could play an important role in wide range of systems, for example, in controlling and enhancing charge transport at interfaces [12] , [38] , in influencing crystal growth [17] or the stability of colloidal solutions and emulsions [18] . In addition, this effect could also be exploited in the design and self-assembly of nanomaterials [39] and used to template nanostructures [16] . Atomic force microscopy Recently, we showed that amplitude-modulation AFM could derive quantitative information about the local free solvation energy of a solid fully immersed into a liquid, with sub-nanometre resolution [31] . This is possible when the vibrating AFM tip dissipates most of its energy within the interfacial liquid, without significant interaction between the tip and the solid [30] , [31] . In this regime, hereafter referred to as ‘interfacial dissipation microscopy’ (IDM), information about the local interfacial energy is contained in the phase image, acquired simultaneously with the topography image of the interface and is related to the local dynamics of the liquid probed by the tip [40] , [41] . When ions adsorb at the surface of the solid, they induce a substantial perturbation of the local solvation environment, which can be detected at the single-ion level by IDM as the AFM tip forces the liquid around the imaged ion [35] . Single Rb + ions can be clearly identified in the topographic IDM images ( Fig. 1a ). The adsorbed Rb + ions appear as distinct protrusions on the sites normally occupied by K + ions in bulk mica (hereafter called ‘binding sites’, Fig. 1b ). In the associated phase image, the ions induce a sharp dark contrast, indicating an increase of the local tip energy dissipation (see also Supplementary Figs 1 and 2 ). 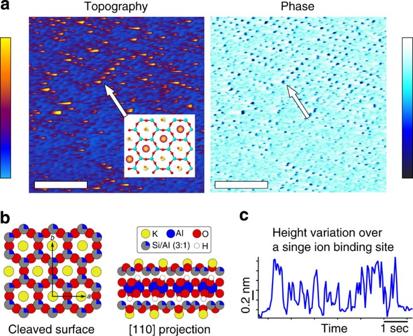Figure 1: IDM imaging of Rb+ions adsorbed at the surface of mica in an aqueous solution. The solution contains 3 mM RbCl. Individual ions can be distinguished both in topography and in phase (a, arrow), often forming geometrical domains or rows. Occasionally, a bright ‘tail’ is visible adjacent to the dark spots attributed to adsorbed ions. This tail is induced by a momentary increase of the tip vibration amplitude as the feedback loop completes its correction, and is due to the particularly gentle imaging conditions. The atomic structure of mica evidences the position of the ion binding sites, which are occupied by K+ions in the bulk crystal (b). Repeatedly scanning over a same binding site (c) yields substantial height variations in time as single Rb+ions adsorb and desorb from the site (see alsoSupplementary Fig. 3). Scale bar, 3 nm (a), and the colour bars represent 1 nm (topography) and 15° (phase). Figure 1: IDM imaging of Rb + ions adsorbed at the surface of mica in an aqueous solution. The solution contains 3 mM RbCl. Individual ions can be distinguished both in topography and in phase ( a , arrow), often forming geometrical domains or rows. Occasionally, a bright ‘tail’ is visible adjacent to the dark spots attributed to adsorbed ions. This tail is induced by a momentary increase of the tip vibration amplitude as the feedback loop completes its correction, and is due to the particularly gentle imaging conditions. The atomic structure of mica evidences the position of the ion binding sites, which are occupied by K + ions in the bulk crystal ( b ). Repeatedly scanning over a same binding site ( c ) yields substantial height variations in time as single Rb + ions adsorb and desorb from the site (see also Supplementary Fig. 3 ). Scale bar, 3 nm ( a ), and the colour bars represent 1 nm (topography) and 15° (phase). Full size image The IDM images reveal interesting peculiarities about the Rb + ions apparent dynamics and organization at the surface of mica. First, the adsorbed Rb + ions appear surprisingly stable, with the same protrusion often visible in several consecutive line scans. Theory [42] and scanning polarization microscopy measurements of ions mobility on mica [43] suggest that the residence time of adsorbed ions at a given binding site should not exceed microseconds, but our IDM measurements of the residence time of Rb + ions over a single binding site ( Fig. 1c ) indicate an average time in the order of 100 ms (see Supplementary Fig. 3 ). However, the result is likely to be limited by the time-resolution capability of IDM measurements (~50 ms), which may probe ionic densities instead of single ions. Nonetheless, the protrusions unambiguously indicate the presence of Rb + ions at the corresponding sites, as evidenced when varying bulk ionic concentration ( Fig. 2b and Supplementary Fig. 4 ). 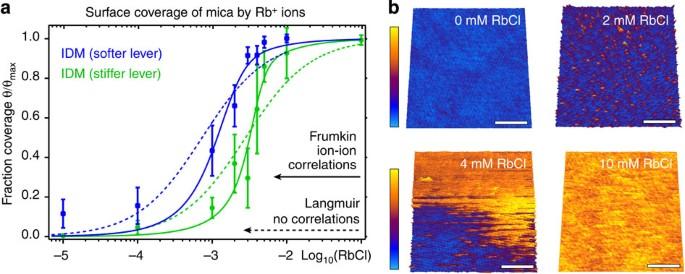Figure 2: Adsorption isotherm of Rb+ions at the surface of mica measured by IDM in solution. The isotherms (a) comprise measurements conducted with two types of cantilevers that exhibit different spring constants (ks~0.1 N m−1for the softer lever andks~0.5 N m−1for the stiffer lever) but a same tip design. The solid lines represent data fits with the Frumkin isotherm, which allows for ion–ion correlations. The dashed lines provide fits without correlations (Langmuir isotherm) (seeSupplementary Methodsfor details). The apparent surface coverage derived from IDM measurements with the softer cantilever is larger than for the stiffer cantilever, consistent with the expected smaller mechanical perturbation (and hence smaller) of the Stern layer by the softer cantilever. The results indicate a relatively small mechanical perturbation energy by the measuring IDM tip (kJ mol−1for the softer lever,Supplementary Fig. 11) but a substantially larger electrostatic perturbation of~7 kJ mol−1for both cantilevers. Control experiments with gold-coated tips confirm the dominance of the electrostatic perturbation (Supplementary Fig. 5). Representative topographic images of the IDM measurements are shown inbfor the stiffer lever (see alsoSupplementary Fig. 4andSupplementary Methodsfor a full set of data). Scale bar, 5 nm (b). Figure 2: Adsorption isotherm of Rb + ions at the surface of mica measured by IDM in solution. The isotherms ( a ) comprise measurements conducted with two types of cantilevers that exhibit different spring constants ( k s ~0.1 N m −1 for the softer lever and k s ~0.5 N m −1 for the stiffer lever) but a same tip design. The solid lines represent data fits with the Frumkin isotherm, which allows for ion–ion correlations. The dashed lines provide fits without correlations (Langmuir isotherm) (see Supplementary Methods for details). The apparent surface coverage derived from IDM measurements with the softer cantilever is larger than for the stiffer cantilever, consistent with the expected smaller mechanical perturbation (and hence smaller ) of the Stern layer by the softer cantilever. The results indicate a relatively small mechanical perturbation energy by the measuring IDM tip ( kJ mol −1 for the softer lever, Supplementary Fig. 11 ) but a substantially larger electrostatic perturbation of ~7 kJ mol −1 for both cantilevers. Control experiments with gold-coated tips confirm the dominance of the electrostatic perturbation ( Supplementary Fig. 5 ). Representative topographic images of the IDM measurements are shown in b for the stiffer lever (see also Supplementary Fig. 4 and Supplementary Methods for a full set of data). Scale bar, 5 nm ( b ). Full size image Second, the ions do not adsorb randomly on the surface of mica, but rather appear to form small islands or rows (arrow in Fig. 1a ) instead of adopting a two-dimensional gas-like random arrangement. This behaviour is confirmed by a statistically significant excess of nearest neighbours for each adsorbed ion, when compared with the same number of ions arranged randomly ( P <0.01, Supplementary Methods ). The result indicates attractive ion–ion interactions, something surprising given the equivalence of the binding sites and the expected electrostatic repulsion between adjacent cations on the surface. This form of attractive interaction is responsible for the observed ion–ion correlation effects, and is at the centre of this study. To better quantify this correlation, we performed IDM measurements of the apparent surface coverage of Rb + ions on mica, as a function of the RbCl bulk concentration in the aqueous solution (see Supplementary Methods for the coverage analysis). These measurements provide Rb + adsorption isotherms from which it is possible to extract the adsorption free energy of the ions to the surface and the correlation energy E c between adjacent ions, using appropriate models [44] , [45] . Practically, any accurate IDM measurement requires first quantification of the effect of the IDM tip on the observed Rb + surface coverage. The tip is charged in water [46] and hence prone to electrostatic interactions with adsorbed ions. In addition, the vibrating tip mechanically perturbs the Stern layer and may displace or remove adsorbed ions. Both these perturbations can artificially change the observed Rb + surface coverage. It is possible to quantify the energies and associated with, respectively, the electrostatic and mechanical perturbations induced by the IDM tip, and hence infer the properties of the unperturbed interface while retaining the IDM imaging resolution. This task is achieved by varying the mechanical perturbation in a quantifiable manner while keeping the electrostatic perturbation constant, using cantilevers with different stiffness but same tip design ( Fig. 2a , Supplementary Fig. 5 and Supplementary Methods ). Control experiments were also conducted with gold-coated tips ( Supplementary Fig. 6 ). Representative images of the IDM measurements for selected bulk RbCl concentrations are shown in Fig. 2b . Assuming that the large majority of Rb + ions are adsorbed in the inner-sphere hydration state at the surface of mica [21] , [47] the IDM-derived isotherms can be fitted with two main models. The simplest model, the Langmuir isotherm [44] , assumes a uniform and homogenous Stern layer with no interactions between adsorbing ions, and therefore the correlation energy ( E c ≡0) is zero (dashed line in Fig. 2a ). Alternatively, a modified Frumkin [45] isotherm model that takes into account both ion–ion correlations and contributions of the IDM tip perturbation, provides a substantially better fit to the data (solid line in Fig. 2a and Supplementary Methods ). The maximum coverage observed by IDM (10 mM, Fig. 2b ) corresponds to all the available binding sites being occupied and the isotherm is modelled accordingly. In reality, only half the binding sites should, on average, be occupied to ensure electro-neutrality at equilibrium [48] . This suggests that at 10 mM, the IDM images predominantly Rb + patches with empty area outside the imaging region. The existence of patches is consistent with correlations effects, and patches are likely to assemble in the vicinity of the negatively charged tip. The observed full surface coverage could also be explained by co-adsorption of Cl − anions, known to occur for Cs + on mica [49] . Co-adsorption is however unlikely to take place here [48] , [50] , also in light of our simulation results ( Supplementary Methods ). The main result from the isotherm analysis is the clear correlation between Rb + ions during the adsorption process. The associated correlation energy was found to be always attractive and similar, within uncertainty, for both types of cantilever E c =−7±3 kJ mol −1 ( Supplementary Methods ). This value is consistent with the observed formation of Rb + rows and small domains at low salt concentration in the IDM images ( Fig. 1 ) and with statistical analysis of number of nearest neighbours ( Supplementary Methods ). In addition, the fact that E c is independent of the magnitude of the IDM perturbation indicates that the correlation is an intrinsic property of the interface. Time-dependent adsorption studies, such as that presented in Fig. 1c , also showed preferential adsorption of ions on several adjacent sites simultaneously ( Supplementary Fig. 3 ), supporting the idea that Rb + –Rb + correlation effects stabilize the Stern layer. This correlation can have two possible origins, either direct electrostatic interactions between adsorbed ions or hydration effects. Electrostatic correlation are known to play an important role in systems with high charge density [51] such as multivalent ions on DNA [52] , but they are unlikely to play a significant role here due to the low charge density of the ions involved. A simple estimate of the electrostatic energy gained by two isolated Rb + ions brought side by side on the surface of mica suggests that some other form of correlation must be taking place ( Supplementary Discussion ). We propose instead that the correlation is induced by a better coordination of the water molecules in the global hydration structure of neighbouring ions, compared with the hydration shell of single adsorbed ions. Under this hypothesis, although electrostatic interactions occur between solvent molecules, ions and the surface, the correlation is effectively controlled by the structural organization of water molecules at the interface. To test this hypothesis, we conducted MD simulations so as to obtain a full molecular-level picture of the Rb + ions dynamics at the surface of mica in water. MD simulations A ‘free’ interface (that is without the presence of an IDM probe) was used in the simulation to assess whether or not the IDM observations reflect the ‘unperturbed’ interface. Owing to limited computational power, current simulations cannot directly replicate IDM experiments in terms of duration or system size. We therefore decided to compare the intrinsic stability of different geometrical configurations for adsorbed ions at the surface of mica in water. Three starting configurations were studied, progressively increasing the average number of direct neighbours between ions: (i) with the cations randomly distributed at the surface of mica ( Fig. 3a ), (ii) with the cations forming a single row on mica ( Fig. 3b ) and (iii) with the cations grouped in a single hexagonal domain on the surface ( Fig. 3c ). In addition, as hydration forces are expected to play an important role in the correlations effects, we also conducted the simulations with K + ions and Na + ions. The K + ions are generally seen as chaotropic [37] similarly to Rb + ions, but are naturally present in mica. In contrast, Na + ions are kosmotropic and exhibit a smaller primary solvation shell with higher hydration energy than K + and Rb + . The simulations comprise ion–ion and ion–mica electrostatic interactions, as well as hydration interactions between water molecules, ions and mica. An ion located within 4 Å of the mica’s hydroxyl oxygen is considered adsorbed ( Supplementary Methods ). The time-averaged interaction energies of the simulation runs are presented in Fig. 3d for each ion type in the three different starting configurations, always with a similar number of ions. 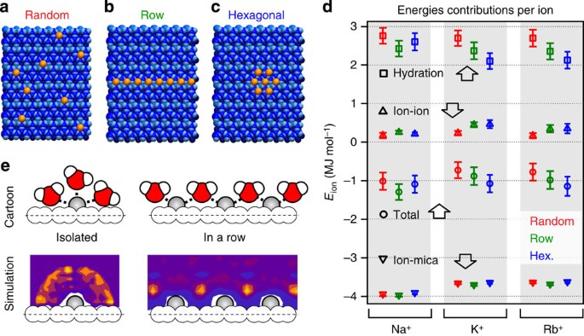Figure 3: Data from the molecular dynamics simulations of mica in aqueous solution. Three different starting configurations have been tested: with the cations randomly adsorbed (a), forming a row on mica (b) or a hexagon (c). The average hydration (open square), electrostatic (open triangles) and total (open circles) free energy of the adsorbed ions is given for each type of ion an each starting configuration (d). The data indare extracted from the evolution of the hydration energy per adsorbed ion throughout the simulation. The error bars indare 2 s.d. Ine, a schematic depiction of the water surrounding adsorbed K+. A clear difference is visible between isolated ions or ions forming geometrical patterns where the location of shared water molecules is well defined. From MD simulations, the density of oxygen atoms of the water molecules is also shown. In the case of single ion, the value of the oxygen density is the radial average around the K+ion. In the case of row of K+, the average oxygen density is obtained by considering a rectangle of 0.5 nm width aligned with the row of the ions and centred on them. Figure 3: Data from the molecular dynamics simulations of mica in aqueous solution. Three different starting configurations have been tested: with the cations randomly adsorbed ( a ), forming a row on mica ( b ) or a hexagon ( c ). The average hydration (open square), electrostatic (open triangles) and total (open circles) free energy of the adsorbed ions is given for each type of ion an each starting configuration ( d ). The data in d are extracted from the evolution of the hydration energy per adsorbed ion throughout the simulation. The error bars in d are 2 s.d. In e , a schematic depiction of the water surrounding adsorbed K + . A clear difference is visible between isolated ions or ions forming geometrical patterns where the location of shared water molecules is well defined. From MD simulations, the density of oxygen atoms of the water molecules is also shown. In the case of single ion, the value of the oxygen density is the radial average around the K + ion. In the case of row of K + , the average oxygen density is obtained by considering a rectangle of 0.5 nm width aligned with the row of the ions and centred on them. Full size image A direct comparison between the simulation runs show that the overall free energy per ion is always higher when adsorbed in random configuration ( Fig. 3d ). Decomposition of this free energy in its hydration (ion–water) and electrostatic (ion–ion and ion–mica) contributions shows that the energy dependence of the ion configuration is largely dominated by the hydration energy. The latter is about an order of magnitude larger than the ion–ion electrostatic potential, and always largest for the random configuration regardless of the type of ions considered. In the case of K + and Rb + , the hydration energy (and the total free energy) per ions decreases with the number of immediate neighbours. However, this trend is not as clear for the Na + ions, mainly due to the particularly high mobility of Na + and the presence of multiple solvation states [47] ( Supplementary Figs 7 and 8 ) leading to a rapid dissolution of the initial geometrical arrangements. This is not the case for K + and Rb + ions, which exist mainly in a single hydration state and tend to remain at the usual ion binding sites when adsorbed [47] . They also exhibit little mobility throughout the simulation ( Supplementary Figs 7 and 8 ), hence allowing for a more direct interpretation of the influence of their adsorption configuration on their respective free energy. One-way analysis of variance of the results demonstrated that the differences in total free energy between geometrical configurations are statistically meaningful for K + and Rb + ( P <0.01). Simulations also show that correlating ions have 10–15% less neighbouring water molecules over the entire length of the simulation compared with randomly adsorbed ions. This shows indirectly the favourability for the entire system to arrange ions on the surface in a correlated way, further supporting hydration as the mechanism driving the local structuring of ions. In Fig. 3e , a simulation snapshot illustrating a possible mechanism is presented. Ions neighbouring each other can share coordinated water molecules and improve the hydration structure compared with a randomly adsorbed ion. Moreover, alternating positive (ions) and negative (water oxygen atoms) charges improves the stability of the structures as predicted by previous theoretical work [53] . The IDM results consistently indicate that the Rb + and K + ions can form ordered structures when adsorbing at the surface of charged crystalline solids in solution. The attractive correlation between neighbouring ions is driven by a better coordination of the surrounding water molecules, as elucidated by the MD simulations. As a result, the effect should depend on the hydration structure of both the adsorbed ion and the surface of the solid. Furthermore, the simulations show that Rb + (and K + ions) prefer to form geometrical arrangements that favour nearest-neighbour configuration between adsorbed ions. Although only a limited number of configurations could be tested, the hexagonal arrangement (3.4 neighbours) appeared consistently more favourable than rows (2 neighbours), with both arrangements preferred over a random adsorption (0 neighbour). This two-dimensional self-assembly process is driven by minimization of the hydration water free energy. MD simulations show that two conditions are necessary for this ordering to take place: the ion’s hydration energy has to dominate over ion–ion electrostatic interactions at the interface, and the hydration properties of the ions considered should allow the formation of a an ordered monolayer, for example, by favouring a single hydration state at the surface of the solid considered. The multiple solvation states of adsorbed Na + ions enable them to move rapidly between different locations not necessarily coinciding with a binding site and embed themselves deeper into the surface ( Fig. 4b and Supplementary Fig. 7 ). The presence of small kosmotropic ions sitting between the main binding sites has already been reported in previous AFM studies [34] and RAXR experiments have also shown that several kosmotropic ions can adsorb in different hydration states simultaneously [47] . The surface of the solid plays an important role in the correlation effects by imposing a set distance between adjacent binding sites. 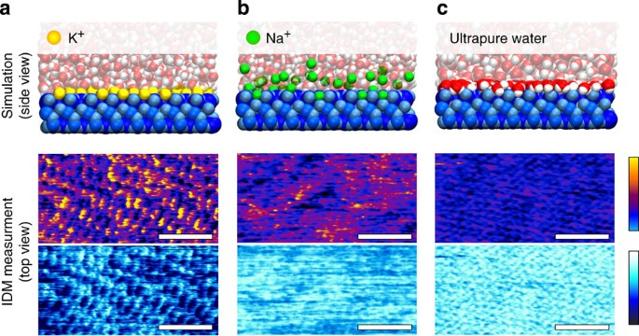Figure 4: Adsorption of K+and Na+ions at the surface of mica seen by simulation and IDM. To allow for a direct comparison, images in K+(a), Na+(b) and water (c) are presented side by side and on a same scale. In each case, a simulation snapshot with semi-transparent water molecules is shown (top) together with the corresponding IDM image (bottom). All the IDM data were acquired with a similar cantilever/tip and in identical operating conditions. The KCl and NaCl bulk concentration are 1 mM and 0.5 mM, respectively, so as to ensure only partial coverage of the mica in each case. The adsorbed ions consistently induce a darker contrast in the phase (as for Rb+), although with a magnitude specific to each ion type. The contrast is less pronounced for Na+ions due to their positions more ‘embedded’ in the mica. The Na+ions sitting further from the surface are only occasionally imaged by the tip. This is also reflected in the smoother topographic image achieved in NaCl. Scale bar, 3 nm (for all images). The colour scale bars are 1 nm (a) and 0.5 nm (b,c) for topography and 30° (a–c) for phase. Figure 4: Adsorption of K + and Na + ions at the surface of mica seen by simulation and IDM. To allow for a direct comparison, images in K + ( a ), Na + ( b ) and water ( c ) are presented side by side and on a same scale. In each case, a simulation snapshot with semi-transparent water molecules is shown (top) together with the corresponding IDM image (bottom). All the IDM data were acquired with a similar cantilever/tip and in identical operating conditions. The KCl and NaCl bulk concentration are 1 mM and 0.5 mM, respectively, so as to ensure only partial coverage of the mica in each case. The adsorbed ions consistently induce a darker contrast in the phase (as for Rb + ), although with a magnitude specific to each ion type. The contrast is less pronounced for Na + ions due to their positions more ‘embedded’ in the mica. The Na + ions sitting further from the surface are only occasionally imaged by the tip. This is also reflected in the smoother topographic image achieved in NaCl. Scale bar, 3 nm (for all images). The colour scale bars are 1 nm ( a ) and 0.5 nm ( b , c ) for topography and 30° ( a – c ) for phase. Full size image To verify experimentally the MD predictions for K + and Na + ions, we obtained IDM images of the surface of mica in KCl and NaCl solutions ( Fig. 4a, b ). The results are fully consistent with the simulations: the K + ions appear similar to Rb + ions, forming domains and rows on the surface and allowing imaging conditions almost as stable as in RbCl (see also Supplementary Fig. 9 and Supplementary Methods ). In contrast, Na + ions appear poorly defined and show no clear structural organization on the surface. Furthermore, the high cations mobility on the surface and the presence of multiple hydration states prevented stable IDM imaging. Interestingly, the phase shift observed for images of K + and Na + is different despite a same cantilever/tip and identical imaging condition. This difference reflects that of the two ions’ hydration shells, suggesting that IDM can even differentiate between adsorbed ions through their specific modification of the interfacial hydration structure. Differences between ions are likely to be enhanced in IDM measurements due to the momentary confinement of the interface by the IDM tip pushing water around the ions’ solvation shell. Previous studies have shown that the hydration structure of a particular ion often dominates its interfacial behaviour under confinement [54] . In IDM measurements, although confinement effects are limited by the small surface of the tip effectively imaging and the slow confining speed (<50 μm s −1 ), they may nonetheless enhance the observations of ion–ion correlations that would otherwise be difficult to capture. Indeed, previous RAXR measurements were unable to detect correlations between Rb + ions within experimental uncertainty [48] . Present MD simulations of the ‘free’ (that is unconfined) interface show that correlations effects constitute an intrinsic property of the system, which we believe is, at best, enhanced by the IDM measurements ( Supplementary Discussion ). To test the generality of our findings, we assessed a final experiment on a different solid: a SAM exposing polar alcohol headgroups (mercaptohexanol, inset Fig. 5 ). The SAM-functionalized gold surface develops a surface potential in aqueous solution. Previous reports indicate zeta-potentials ranging between −40 and −50 mV for gold nanoparticles coated with alcohol-terminated alkanes in an aqueous solution at a similar pH [55] , [56] . The SAM surface potential is weaker than that of mica. Significantly, the SAM surface in direct contact with the liquid is not charged and the polar alcohol groups interact with the liquid mainly through the formation of hydrogen bonds. The surface potential of the SAM can hence be seen as a diffused background, creating an incentive for cations to form an EDL close to the SAM’s surface. The molecular packing of the SAM creates a hydration landscape similar to that of mica at the nanoscale [26] , [57] and ion–ion correlations can be expected to occur. 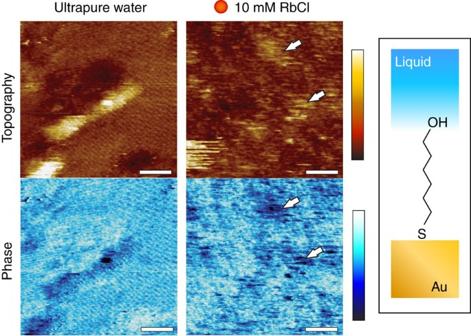Figure 5: IDM images of a mercaptohexonol SAMs in water and in a 10 mM RbCl solution. In both cases, the SAM lattice can be identified. In the presence of the salt, Rb+ions can be seen clustering at the SAM surface (arrows), creating a consistent darker contrast in the phase image. The ion clusters are however easily removed by the scanning tip, making them appear less clearly than on mica due to a weaker attractive interactions with the surface (weaker surface potential). The chemical structure of a mercaptohexanol molecule is illustrated by a cartoon (inset on the right). Scale bars, 4 nm (water) and 3 nm (RbCl), and colour scale bars are 0.7 nm for topography and 20° for phase. Figure 5 compares high-resolution IDM images acquired in ultrapure water and in 10 mM RbCl. In the presence of the salt, Rb + clusters can be identified at the surface of the SAM, yielding a phase contrast consistent with the results on mica. The clusters are however less clearly defined than on mica and can easily be removed by the tip. This can be explained by the relatively weak surface potential of the SAM that limits the incentive for adsorbed ions to remain at the surface. Nonetheless, the results confirm that in the presence of an appropriate hydration landscape, correlated ion clusters can form solely through hydration forces, and that the effect is not limited to mica. Figure 5: IDM images of a mercaptohexonol SAMs in water and in a 10 mM RbCl solution. In both cases, the SAM lattice can be identified. In the presence of the salt, Rb + ions can be seen clustering at the SAM surface (arrows), creating a consistent darker contrast in the phase image. The ion clusters are however easily removed by the scanning tip, making them appear less clearly than on mica due to a weaker attractive interactions with the surface (weaker surface potential). The chemical structure of a mercaptohexanol molecule is illustrated by a cartoon (inset on the right). Scale bars, 4 nm (water) and 3 nm (RbCl), and colour scale bars are 0.7 nm for topography and 20° for phase. Full size image The overall picture emerging from IDM measurements and MD simulations highlights the importance of the interplay between the hydration properties of adsorbed ions and that of the surface for ordering the ions. In the case of mica, chaotropic ions, such as K + or Rb + , appear mostly located within the first hydration layer with limited effect over the distal layers ( Supplementary Figs 7 and 10 ). This minimal disruption of the mica’s interfacial water structure allows the formation of stable ionic structures guided by the particular hydration landscape of mica. The self-assembly takes place within mica’s first hydration layer and is guided by a minimization of the overall hydration energy of both the mica and the adsorbed ions. The resulting correlation effect does not require any specific interaction between the ions and the surface, and can, in principle, occur at any interface that exhibits an appropriate hydration landscape. In addition, the short Bjerrum length of hydrated monovalent ions (~1 nm, Supplementary Discussion ) makes it possible for correlation effects to take place at the surface of solids with lower surface charge density than mica, as illustrated for the SAM. Finally, given the ubiquity of K + ion in biology, this type of water-induced correlation may be commonplace at the surface of biomembranes where gel-phase phospholipid domains tend to adopt an arrangement with a similar periodicity as the mica lattice or the SAM studied here. Biological interfaces are however more complex, due to their strong and local dependence on the surrounding pH, and the conformational flexibility of the molecules. Correlated ionic networks are however likely to play key roles in charge transfer [12] , [38] and membrane shaping [58] , and both experiments and simulations are already underway to examine these possibilities. In this study, we have shown that single metal ions can form ordered structures at solid–liquid interfaces through water-induced correlation effects. The effect, observed experimentally at the single-ion level by IDM, is driven by the interfacial water, and depends on the hydration properties of the ions considered. MD simulations of different types of monovalent ions at the interface with mica highlight the delicate interplay between the hydration structure of the solid and that of the adsorbing ions, and correctly predict the IDM observations. The simplicity of the system and the generality of the effect suggest that it may spontaneously occur in a large variety of systems. Interfacial dissipation microscope All the AFM data were acquired on a Multimode Nanoscope IIIa (Digital Instruments) operated in the IDM regime (see text). The sample and the scanning tip were fully immersed into the imaging solution. Before each experiment, the AFM liquid cell was thoroughly washed by consecutive sonication in isopropanol and ultrapure water, and then dried under nitrogen flow. A cantilever was then mounted on the cell and engaged over clean mica in ultrapure water. After the AFM had reached thermal equilibrium, the ultrapure water was removed and the desired solution was injected into the cell. We used standard silicon nitride cantilevers (Olympus RC800 PSA, Olympus, Tokyo) with two different lever length but identical tip design. The nominal spring constant of the levers were k s =0.1 N m −1 (softer lever) or k h =0.76 N m −1 (stiffer lever). Cantilevers from a same wafer were used to allow for better comparison of the results. The cantilevers were calibrated using their thermal spectra [59] after each experiment and found to have typical stiffness and Q -factors of k h ~0.5 N m −1 and Q h ~4.4 (stiffer lever), and k s ~0.1 N m −1 and Q s ~2.5 (softer lever). The cantilever was driven acoustically in a liquid cell, close to its resonance frequency. Typical working amplitudes A were kept between 0.8 and 1.5 nm with the setpoint ratio A / A 0 as large as possible, where A 0 is the free vibration amplitude of the lever in the liquid far from the mica surface. When operated in these conditions, atomic-level resolution topographic and phase images of the type shown in Figs 1 , 2 and 4 could be routinely achieved. We found that too small amplitudes (<0.5 nm) resulted in no apparent surface coverage by the ions due to the tip ‘sweeping’ the ions sideways. In general, as the IDM tip can mechanically remove ions from the surface (see Fig. 2 ), we always carefully balanced the imaging setpoint so as to keep it as large as possible. Nonetheless, minute setpoint variations were sufficient to introduce variations in the apparent surface coverage; this is the main source of error in our statistical analysis (see Supplementary Methods ). Sample preparation High-quality muscovite mica (grade V) was purchased from SPI supply (West Chester, PA, USA) and used in all the experiments. The mica was freshly cleaved with adhesive tape and rinsed copiously with ultrapure water (18.2 MΩ, Merck Millipore, Billerica, MA, USA) before use. The SAM of mercaptohexanol were created on gold substrates. The substrates, commercially available (PHASIS, Geneva, Switzerland), consisted of gold evaporated on mica, packaged in a sealed nitrogen atmosphere. On opening, the substrates were immediately placed in vials containing 10 ml of ethanolic solution of 6-mercaptohexan-1-ol (mercaptohexanol) (TCI America, Portland, OR, USA). The thiol concentration was 0.01 mM. The substrates were left in the solution in dark at room temperature for a period of 7 days, at which point they were rinsed with ethanol seven times and dried under a gentle argon flow. All the solutions were prepared in ultrapure water with 99.9% pure salts purchased from Sigma-Aldrich and used as received. MD simulations Based on the previously reported crystal structure of muscovite [60] , we constructed for the MD simulations a crystal measuring ~41 × 55 × 40 Å with the (001) plane set parallel to the xy plane of the simulation referential. The exposed plane naturally contains potassium ions, and depending on the required starting configuration all, none or a selected number of these ions were removed or replaced with a different ion species, resulting in either a random, row or hexagon configuration for the surface ions. In all cases, we ensured complete system charge neutrality. This fully atomistic model of muscovite is centred in a periodic simulation box and solvated in the direction perpendicular to the exposed plane, ensuring a water thickness on top of the mica of at least 5 nm. To describe the interactions between all atoms, two force fields are used. For the muscovite mica interactions and all ion interactions, we used the CLAYFF force field [61] , which is a general force field suitable for the simulation of hydrated and multicomponent mineral systems and their interfaces with aqueous solutions. The interactions between water molecules were described by the TIP3P model of the CHARMM force field [62] . Recently, it has been shown that the CLAYFF and CHARMM force fields are compatible and can be used together [63] , [64] , [65] , [66] . All simulations have been performed using the MD code NAMD [67] . For visual inspection, VMD [68] was used and most of the analysis was performed using the Python library MDAnalysis [69] . Three different surface arrangements were examined for each type of ion: (i) a row of ions along the (100) direction, (ii) a hexagon and (iii) ions randomly placed. In the case of the row and the random distributions, eight ions were placed at the surface, while seven ions (a full hexagon) were used in the hexagonal configuration. Examples of these arrangements are depicted in Fig. 3a–c . For each of the nine different MD simulations, a similar protocol is followed. This includes an initial minimization of the energy associated to the water only (allowing bad contacts to be removed), followed by a short dynamics run of 5 ps to equilibrate the entire system at ambient conditions, and finally the production run of 1 ns. Only the latter is used for analysis. The current simulation set-up and protocol is similar to the setup used previously to study the interaction between calcite, water and ions [35] , but in the current work all simulations are performed in duple to improve statistical accuracy and to account for individual aberrations. To verify our muscovite model, we computed basic properties such as water residence time near the muscovite surface and around the ions in solution, as well as the hydration numbers for these ions. We found all of the measured properties to be in good agreement with previously reported data [47] , [49] , [70] . For instance, the hydration numbers computed from our simulations are 5.8, 7.1 and 7.9 for Na + , K + and Rb + , respectively, in bulk water. As rubidium is a less common ion to encounter in mineral force fields such as CLAYFF or organic force fields such as CHARMM, the properties for this ion were checked more carefully and found comparable to experimental values reported [21] , [48] , [50] . How to cite this article : Ricci, M. et al . Water-induced correlation between single ions imaged at the solid–liquid interface. Nat. Commun. 5:4400 doi: 10.1038/ncomms5400 (2014).